Nasal immunity is an ancient arm of the mucosal immune system of vertebrates The mucosal surfaces of all vertebrates have been exposed to similar evolutionary pressures for millions of years. In terrestrial vertebrates such as birds and mammals, the nasopharynx-associated lymphoid tissue (NALT) represents a first line of immune defence. Here we propose that NALT is an ancient arm of the mucosal immune system not restricted to terrestrial vertebrates. We find that NALT is present in rainbow trout and that it resembles other teleost mucosa-associated lymphoid tissues. Trout NALT consists of diffuse lymphoid cells and lacks tonsils and adenoids. The predominant B-cell subset found in trout NALT are IgT + B cells, similar to skin and gut. The trout olfactory organ is colonized by abundant symbiotic bacteria, which are coated by trout secretory immunoglobulin. Trout NALT is capable of mounting strong anti-viral immune responses following nasal delivery of a live attenuated viral vaccine. Our results open up a new tool for the control of aquatic infectious diseases via nasal vaccination. Olfaction is one of the most ancient sensory systems and is vital for all animals. In terrestrial vertebrates, the olfactory system detects low concentrations of airborne, volatile chemical substances, whereas aquatic vertebrates, such as teleost fish, encounter waterborne odorants. Strikingly, the sensory systems of ancient aquatic vertebrates are anatomically similar to the olfactory systems of land-based animals. Thus, the conservation of olfactory systems in a broad array of animals implies that there is an optimal solution to the problem of detecting and discriminating odours [1] . The nasopharynx-associated lymphoid tissue (NALT) was first discovered in rodents as a paired mucosal lymphoid organ, located on the roof of the soft palate, at the entrance of the pharyngeal duct [2] . Currently, NALT is considered the first line of defence against airborne antigens and so far has only been described in birds and mammals. Thus, evolutionary speaking, NALT is thought to have emerged circa 200 million years ago when the first mammals appeared. However, the olfactory system of aquatic vertebrates must be able to fight waterborne antigens and is subject to similar evolutionary forces than that of terrestrial vertebrates. We hypothesize that olfaction and immunity represent an ancient association in the vertebrate lineage and is present in ancient aquatic vertebrates. The latter breaks the current paradigm that regards NALT as strictly present in terrestrial vertebrates. Teleost fish represent the most ancient bony vertebrates with a dedicated mucosal immune system [3] . Three different mucosa-associated lymphoid tissues (MALTs) have been characterized in teleosts thus far: gut-associated lymphoid tissue (GALT), skin-associated lymphoid tissue and gill-associated lymphoid tissue [4] . Importantly, all three MALT share a number of conserved features. The common canonical features of all teleost MALT are: (i) the presence of diffuse lymphoid cells with the absence of organized lymphoid structures; (ii) a predominant role for IgT antibodies (the specialized mucosal immunoglobulin class in teleosts) and IgT + B cells [5] , [6] ; (iii) the presence of a diverse microbial community and coating of commensals by mucosal Igs. The presence of common canonical features found in all three types of teleost MALT suggests that these may also be conserved in teleost NALT. In order to gain further insights into the origins of nasal immunity in vertebrates, we investigate here the main immune players and immune responses present in the olfactory organ of an ancient vertebrate, the rainbow trout ( Oncorhynchus mykiss ). Our studies show that teleost NALT is broadly similar to other MALT previously described in fish. Furthermore, we demonstrate that the rainbow trout olfactory system is capable of mounting strong innate and adaptive immune responses. Finally, we show that nasal vaccination is a very effective and novel tool for the control of both viral and bacterial aquatic infectious diseases in fish. Teleost NALT shares canonical features with teleost MALT Teleost gut, skin and gills contain diffuse lymphoid cells but lack any organized lymphoid structures such as those found in mammals. In order to understand the histological organization of teleost NALT, we examined formalin-fixed olfactory organs stained with either toluidine blue or haematoxylin/eosin obtained from four different teleost families: Polyprionidae (Order Perciforms); Salmonidae (Order Salmoniforms); Cyprinidae (Order Cypriniforms) and Anguillidae (Order Anguilliformes; Fig. 1a–d ). Despite some minor morphological differences, the olfactory rosettes of New Zealand groper ( Polypryon oxygeneios ), rainbow trout ( O. mykiss ), goldfish ( Carassius auratus ) and Australian eel ( Anguilla australis ) all harbour abundant myeloid and lymphoid cells scattered intraepithelially (IELs) as well as in the lamina propria leucocytes (LPLs; Fig. 1a–d ). This distribution was conserved in all four species and resembles the teleost GALT, where two populations, IELs and LPLs, are known to be present. It has been previously shown that in mucosal lymphoid tissues such as the gut and the skin, IgT + B cells contribute to 50–60% of the total B cells, compared with systemic lymphoid organs where they are only ~25% of the total B cells [5] , [6] . Here, we isolated the leucocytes from the olfactory organ of adult rainbow trout and studied the abundance of IgT + and IgM + B cells by flow cytometry using specific monoclonal antibodies. We found that, similar to the gut, IgT + B cells make up ~51.5% of the total B cells in the olfactory organ of rainbow trout, whereas ~48.5% of the B cells are IgM + ( Fig. 1e,f ). We next performed immunofluorescence staining to determine where IgT + and IgM + B cells are located in the trout olfactory organ. We found that both B-cell types were present mostly within the epithelial layer ( Fig. 1g ) and not the LP ( Supplementary Fig. 1 ) unlike in the gut where they are predominantly located in the LP. Mucosal IgM and IgT are transported across epithelia via the polymeric Ig receptor (pIgR) [5] , [6] . Using a polyclonal anti-trout pIgR antibody, we found abundant pIgR staining at the apical areas of the mucosal epithelium of the trout olfactory organ indicating that this receptor is a mechanism by which Igs reach the lumen of the nasal cavity of trout ( Fig. 1h ). Finally, the mucosal secretions of trout skin and gut are characterized by having a higher IgT to IgM concentration ratio than that in serum [5] , [6] . Using immunoblot, we measured the IgT/IgM protein levels in the nasal mucus and serum of rainbow trout. The nasal mucus samples used in this experiment were devoid of bacteria as bacteria were removed before performing immunoblots. Therefore, we measured the levels of free Igs as opposed to total Ig levels, which would include both free Igs and Igs coating bacteria. The IgT/IgM ratio in nasal mucus was ~20 times that of serum ( Fig. 1i ). This value is lower than previously reported values in skin and gut mucus (37 and 64 times, respectively) because of the fact that those studies used total mucus samples. 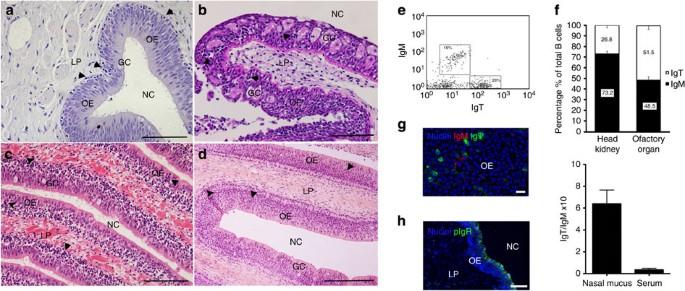Figure 1: General organization of teleost NALT. The olfactory organ of four different families of teleost fish harbours diffuse lymphoid cells but lacks organized NALT. (a) Toluidine blue stain of the olfactory organ of a control adult rainbow trout (O. mykiss). (b) Haematoxylin/eosin stain of the olfactory organ of a control adult goldfish (C. auratus). (c) Haematoxylin/eosin stain of the olfactory organ of a control adult New Zealand groper (P. oxygeneios). (d) Haematoxylin/eosin stain of the olfactory organ of a control adult Australian eel (A. australis). Arrowheads indicate lymphocytes. GC, goblet cells; LP, lamina propria; NC, nasal cavity; OE, olfactory epithelium. Scale bar, 100 μm. (e) Flow cytometry analysis of rainbow trout NALT leukocytes stained with anti-IgM and anti-IgT antibodies. Numbers in outlined boxes indicate the percentage of IgM+(top left) and IgT+(bottom right) B cells. (f) Frequency (mean±s.e.) IgM+and IgT+cells among all B cells present in control rainbow trout NALT (N=15). (g) Immunofluorescence staining for IgM (red) and IgT (green) in a cryosection of rainbow trout olfactory organ (N=5); nuclei (blue) are stained with the DNA-intercalating dye DAPI. Scale bar, 10 μm. (h) Immunofluorescence staining for pIgR (green) in a cryosection of rainbow trout olfactory organ (N=5). Nuclei (blue) are stained with the DNA-intercalating dye DAPI. Scale bar, 100 μm. (i) Mean ratio of IgT to IgM in nasal mucus and serum (N=4) calculated by immunoblotting. Figure 1: General organization of teleost NALT. The olfactory organ of four different families of teleost fish harbours diffuse lymphoid cells but lacks organized NALT. ( a ) Toluidine blue stain of the olfactory organ of a control adult rainbow trout ( O. mykiss ). ( b ) Haematoxylin/eosin stain of the olfactory organ of a control adult goldfish ( C. auratus ). ( c ) Haematoxylin/eosin stain of the olfactory organ of a control adult New Zealand groper ( P. oxygeneios ). ( d ) Haematoxylin/eosin stain of the olfactory organ of a control adult Australian eel ( A. australis ). Arrowheads indicate lymphocytes. GC, goblet cells; LP, lamina propria; NC, nasal cavity; OE, olfactory epithelium. Scale bar, 100 μm. ( e ) Flow cytometry analysis of rainbow trout NALT leukocytes stained with anti-IgM and anti-IgT antibodies. Numbers in outlined boxes indicate the percentage of IgM + (top left) and IgT + (bottom right) B cells. ( f ) Frequency (mean±s.e.) IgM + and IgT + cells among all B cells present in control rainbow trout NALT ( N =15). ( g ) Immunofluorescence staining for IgM (red) and IgT (green) in a cryosection of rainbow trout olfactory organ ( N =5); nuclei (blue) are stained with the DNA-intercalating dye DAPI. Scale bar, 10 μm. ( h ) Immunofluorescence staining for pIgR (green) in a cryosection of rainbow trout olfactory organ ( N =5). Nuclei (blue) are stained with the DNA-intercalating dye DAPI. Scale bar, 100 μm. ( i ) Mean ratio of IgT to IgM in nasal mucus and serum ( N =4) calculated by immunoblotting. Full size image Trout olfactory organ harbours a bacterial community coated by mucosal Igs Teleost are known to have diverse microbial communities that colonize the skin, gut and gill mucosal surfaces. Here we performed 16 s fluorescent in situ hybridization using universal 16 s probes and found the presence of bacteria associated with the olfactory epithelium of trout ( Fig. 2a,b ). Using previously published methods [5] , [6] , we isolated the nasal-associated bacteria and immunostained them with anti-IgM and anti-IgT antibodies in order to measure levels of coating by trout Igs. In trout gut and skin, a predominant percentage of commensal bacteria are coated with IgT [5] , [6] . The presence of high amounts of Igs in the nasal mucosal secretions of trout led us to hypothesize that nasal Igs might also be coating nasal bacteria. We found that ~34% of the nasal-associated bacteria are uncoated and ~66% are coated by mucosal Igs ( Fig. 2h ). These values are consistent with previous findings in the gut (~28% uncoated and ~72% coated) and the skin (~40% uncoated and ~60% coated) [5] , [6] . In the olfactory organ, we found that out of the coated bacteria, ~34% are double coated, ~16% are coated with IgM and ~16% with IgT ( Fig. 2c–g ). This distribution differs from that of gut and skin bacteria where a majority of bacteria are coated by IgT [5] , [6] . Immunoblotting further confirmed that trout nasal-associated bacteria are coated with both mucosal IgT and IgM ( Fig. 2f ). 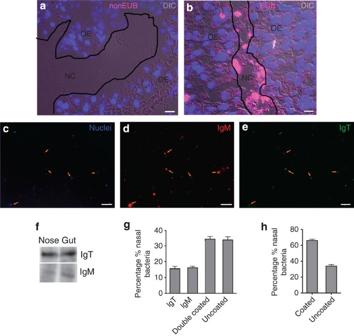Figure 2: Trout nasal bacteria are coated by secretory immunoglobulins. (a) Differential interference contrast images of trout olfactory organ stained with NONEUB oligoprobe by fluorescencein situhybridization. Note that no bacterial staining was observed (N=5). (b) Differential interference contrast images of trout olfactory organ stained with EUB338 oligoprobe (magenta) that stains ~90% of all eubacteria. Abundant bacteria (magenta) can be observed in the lumen of the olfactory organ and some within the olfactory epithelium (N=5). Nuclei (blue) are stained with the DNA-intercalating dye DAPI. Scale bar, 20 μm. (c–e) Fluorescent microscopy images of trout nasal bacteria stained with a DAPI-Hoeschst solution (blue;c), anti-IgM (red;d) or anti-IgT (green;e). Orange arrows indicate bacteria that are positive for DAPI, IgM and IgT (double-coated population). Scale bar, 20 μm. (f) Immunoblot analysis of IgT and IgM on nasal-associated bacteria and gut luminal bacteria (as a positive control). (g) Percentage of trout nasal-associated bacteria that are uncoated, coated with IgT, IgM or both IgT and IgM quantified from immunofluorescence microscopy images. (h) Percentage of trout nasal-associated bacteria that are uncoated or coated with at least one antibody isotype quantified from immunofluorescence microscopy images. Data (mean±s.e.) are representative of three independent experiments (N=6). Figure 2: Trout nasal bacteria are coated by secretory immunoglobulins. ( a ) Differential interference contrast images of trout olfactory organ stained with NONEUB oligoprobe by fluorescence in situ hybridization. Note that no bacterial staining was observed ( N =5). ( b ) Differential interference contrast images of trout olfactory organ stained with EUB338 oligoprobe (magenta) that stains ~90% of all eubacteria. Abundant bacteria (magenta) can be observed in the lumen of the olfactory organ and some within the olfactory epithelium ( N =5). Nuclei (blue) are stained with the DNA-intercalating dye DAPI. Scale bar, 20 μm. ( c – e ) Fluorescent microscopy images of trout nasal bacteria stained with a DAPI-Hoeschst solution (blue; c ), anti-IgM (red; d ) or anti-IgT (green; e ). Orange arrows indicate bacteria that are positive for DAPI, IgM and IgT (double-coated population). Scale bar, 20 μm. ( f ) Immunoblot analysis of IgT and IgM on nasal-associated bacteria and gut luminal bacteria (as a positive control). ( g ) Percentage of trout nasal-associated bacteria that are uncoated, coated with IgT, IgM or both IgT and IgM quantified from immunofluorescence microscopy images. ( h ) Percentage of trout nasal-associated bacteria that are uncoated or coated with at least one antibody isotype quantified from immunofluorescence microscopy images. Data (mean±s.e.) are representative of three independent experiments ( N =6). Full size image Trout olfactory organ expresses immune genes at the steady state To understand whether or not the olfactory organ of rainbow trout expresses immune relevant genes in the absence of antigenic stimulation, we first measured the levels of expression of several immune genes and a number of markers for the main myeloid and lymphoid cells types. Reverse transcription quantitative real-time PCR (RT-qPCR) was used to compare expression levels in control adult rainbow trout olfactory organ to expression levels present in the head-kidney (HK), the major lymphoid organ in teleosts, and muscle, a control non-lymphoid tissue. The olfactory receptor 2 served as a positive control gene for the olfactory organ. We found that most immune markers studied were expressed at similar levels in the olfactory organ and the HK, indicating the previously unrealized but key immunological function of the olfactory organ in rainbow trout ( Fig. 3 , primers used are shown in Supplementary Table 1 ) even in the absence of antigenic stimulation. 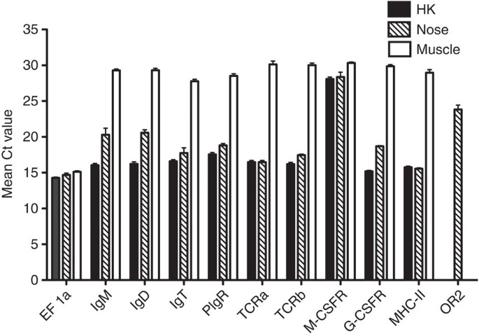Figure 3: Basal expression of immune markers in trout NALT. Expression levels in most cases are comparable to those of the head-kidney (HK), the main haematopoietic organ in teleosts. Quantitative real-time PCR of mRNAs for immune markers in trout HK, OO and muscle (N=6). Data are expressed as mean Ct values±s.e. G-CSFR, granulocyte colony stimulating factor receptor; M-CSFR, macrophage colony stimulating factor receptor; ND, not detected; OR-2, olfactory receptor 2; OO, olfactory organ; TCRb, T-cell receptor beta; TRCa, T-cell receptor alpha. Figure 3: Basal expression of immune markers in trout NALT. Expression levels in most cases are comparable to those of the head-kidney (HK), the main haematopoietic organ in teleosts. Quantitative real-time PCR of mRNAs for immune markers in trout HK, OO and muscle ( N =6). Data are expressed as mean Ct values±s.e. G-CSFR, granulocyte colony stimulating factor receptor; M-CSFR, macrophage colony stimulating factor receptor; ND, not detected; OR-2, olfactory receptor 2; OO, olfactory organ; TCRb, T-cell receptor beta; TRCa, T-cell receptor alpha. Full size image Trout nasal immunization elicits strong local immune responses We next evaluated the effects of intranasal delivery (IN) of a live attenuated viral vaccine against infectious haematopoietic necrosis virus (IHNV). IHNV is a fatal Novirhabdovirus that threatens salmonid species including rainbow trout, Chinook salmon ( O. tshawytscha) , sockeye salmon ( O. nerka ) and Atlantic salmon ( Salmo salar ) worldwide [7] . The selection of this model was based on previous works that had showed the importance of the olfactory organ as infection site for IHNV in salmonids [8] , as well as evidence for some IHNV strains to have neurotropic manifestations [9] . Both reports pointed to the high likelihood of a live attenuated IHNV vaccine to be uptaken by the olfactory organ of salmonid fish and elicit an immune response. To gain some insights on the kinetics of the immune responses that takes place following IN immunization, the olfactory organ and HK of trout that received the IHNV vaccine IN and control trout (PBS) were sampled at days 1, 4, 7, 14, 21 and 28. Thirteen immune relevant genes and cell markers were measured by RT-qPCR. These preliminary studies show that following IHNV vaccine delivery into the olfactory cup, trout mount an immune response both in the HK (systemic; Fig. 4a ) and olfactory organ (local; Fig. 4b ). Importantly, days 4 and 14 were the most relevant in terms of the intensity of the immune response ( Fig. 4 ) and therefore these two time points were selected for subsequent oligo-microarray analysis where the expression of a total of 44K features was analysed. All microarray results were validated by measuring the expression of six candidate genes (three that were upregulated and three that were downregulated in the microarray) by RT-qPCR ( Supplementary Fig. 2 ). The expression of a total of 8,556 (day 4) and 2,228 (day 14) genes were significantly modified following nasal vaccine delivery, with 4,216 and 1,315 genes upregulated, and 4,348 and 913 genes downregulated at days 4 and 14, respectively ( Fig. 5a and Supplementary Tables 2 and 3 ). To further understand the transcriptomic data, we carried out a gene ontology (GO) enrichment to determine the biological processes that were significantly altered following nasal vaccination. This overview indicated that biological processes representing genes involved in protein metabolism, immune response, cell proliferation and apoptosis, and nervous and circulatory system development ( Fig. 5b,c ) were all over represented in the differentially expressed set of genes. Among the genes that play a central role in the nasal immune response, we found on day 4 a significant modification in expression of: (i) genes involved in innate immunity ( Fig. 5d ; such as interleukins, interferons, chemokines, complement factors, mucins, antimicrobial peptides, Toll-like receptors and immunoproteasome subunits); (ii) adaptive immunity ( Fig. 3e ; including MHC complex genes, B- and T-cell receptors and Igs; (iii) antiviral genes ( Fig. 5f ; that is, Mx, TLR3); (iv) NALT-related genes ( Fig. 5g ; C–C motif chemokine 19 (CCL19), L-selectin, vascular cell adhesion protein 1, integrin alpha-M, carbohydrate sulfotransferase 1, C–C motif chemokine 28) and (v) oxidative stress-related genes (that is, heat-shock proteins and glutathione peroxidase). In addition, the expression of some neuronal and olfactory-related genes was also significantly upregulated in response to IHNV IN vaccine. 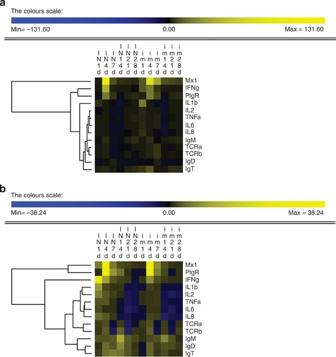Figure 4: Kinetics of the immune response following nasal or injection vaccination. Heat map illustrates results from quantitative real-time PCR of mRNAs for selected immune markers in IHNV-immunized fish versus control fish measured at 1, 4, 7, 14, 21 and 28 days post vaccination (N=6) in the head-kidney (HK;a) and local immune response in the olfactory organ (b) of rainbow trout. Data are expressed as mean fold increase in expression±s.e. qPCR measurements were analysed by unpairedt-test, withP-values <0.05 considered significant. Figure 4: Kinetics of the immune response following nasal or injection vaccination. Heat map illustrates results from quantitative real-time PCR of mRNAs for selected immune markers in IHNV-immunized fish versus control fish measured at 1, 4, 7, 14, 21 and 28 days post vaccination ( N =6) in the head-kidney (HK; a ) and local immune response in the olfactory organ ( b ) of rainbow trout. Data are expressed as mean fold increase in expression±s.e. qPCR measurements were analysed by unpaired t -test, with P -values <0.05 considered significant. 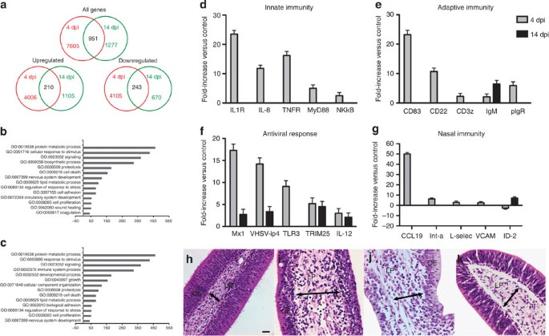Figure 5: Microarray studies of the olfactory organ of rainbow trout. (a) Venn diagrams of microarray experiment representing the overlap of genes upregulated or downregulated in the olfactory organ of rainbow trout 4 or 14 days after IN vaccination with IHNV versus control fish. (b) Biological processes that were significantly altered following the IN vaccination 4 d.p.i. revealed by microarray studies. (c) Biological processes that were significantly modified following the IN vaccination 14 d.p.i. revealed by microarray studies. Fold change differences between control and IHNV-injected samples were calculated using cutoff of twofold. Significant differential expression at each time point (4 and 14 d.p.i.) was established by two sample (unpaired)t-tests (P<0.05) with unequal variance. (d) Representative innate immune genes modulated by IHNV vaccination at 4 or 14 d.p.i. (e) Representative adaptive immune gene expression modulated IHNV vaccination at 4 or 14 d.p.i. (f) Representative antiviral response genes expression modulated by IHNV vaccination at 4 or 14 d.p.i. (g) NALT-related genes differentially up- or downregulated in the olfactory organ of rainbow trout following nasal IHNV vaccination at 4 or 14 d.p.i. (h) Histology of the olfactory epithelium of a mock-vaccinated rainbow trout (N=4). (i) Histological examination (haematoxylin/eosin stain) of the olfactory organ of IN vaccinated rainbow trout 4 d.p.i. with IHNV vaccine (N=4). (j) Histological examination (haematoxylin/eosin stain) of the olfactory organ of IN IHNV-vaccinated rainbow trout 14 d.p.i. (N=4). (k) Histological examination (haematoxylin/eosin stain) of the olfactory organ of IN IHNV-vaccinated rainbow trout 28 d.p.i. (N=4). Scale bar, 10 μm. Black arrows indicate the width of the lamina propria (LP). OE, olfactory epithelium. The red asterisk denotes capillaries in the LP of IN vaccinated trout. Full size image Figure 5: Microarray studies of the olfactory organ of rainbow trout. ( a ) Venn diagrams of microarray experiment representing the overlap of genes upregulated or downregulated in the olfactory organ of rainbow trout 4 or 14 days after IN vaccination with IHNV versus control fish. ( b ) Biological processes that were significantly altered following the IN vaccination 4 d.p.i. revealed by microarray studies. ( c ) Biological processes that were significantly modified following the IN vaccination 14 d.p.i. revealed by microarray studies. Fold change differences between control and IHNV-injected samples were calculated using cutoff of twofold. Significant differential expression at each time point (4 and 14 d.p.i.) was established by two sample (unpaired) t -tests ( P <0.05) with unequal variance. ( d ) Representative innate immune genes modulated by IHNV vaccination at 4 or 14 d.p.i. ( e ) Representative adaptive immune gene expression modulated IHNV vaccination at 4 or 14 d.p.i. ( f ) Representative antiviral response genes expression modulated by IHNV vaccination at 4 or 14 d.p.i. ( g ) NALT-related genes differentially up- or downregulated in the olfactory organ of rainbow trout following nasal IHNV vaccination at 4 or 14 d.p.i. ( h ) Histology of the olfactory epithelium of a mock-vaccinated rainbow trout ( N =4). ( i ) Histological examination (haematoxylin/eosin stain) of the olfactory organ of IN vaccinated rainbow trout 4 d.p.i. with IHNV vaccine ( N =4). ( j ) Histological examination (haematoxylin/eosin stain) of the olfactory organ of IN IHNV-vaccinated rainbow trout 14 d.p.i. ( N =4). ( k ) Histological examination (haematoxylin/eosin stain) of the olfactory organ of IN IHNV-vaccinated rainbow trout 28 d.p.i. ( N =4). Scale bar, 10 μm. Black arrows indicate the width of the lamina propria (LP). OE, olfactory epithelium. The red asterisk denotes capillaries in the LP of IN vaccinated trout. Full size image At day 14, microarray analysis showed the absence of inflammatory responses with no proinflammatory cytokines upregulated at this point. The complement factors C4, C3 and C1q, the chemokine CXC9 and some oxidative stress immune genes were still upregulated at this point. Importantly, at day 14, the number of genes involved in the adaptive immune response (Igs) and their level of expression were significantly higher than at day 4, indicating the induction of an adaptive immune response following IN IHNV vaccine delivery ( Fig. 5e ). Rainbow trout have three Ig isotypes: IgM, IgT and IgD [10] , [11] . Although all three Ig heavy chain genes responded to nasal immunization, IgM appears to play a major role in local nasal immunity, at least in the IHNV vaccine model as it was the most significantly upregulated Ig gene. Out of all the NALT-related genes identified at day 4, only CCL19 continued to be significantly upregulated at day 14. CCL19 is a chemokine that controls the organization and function of NALT [12] . Strikingly, the inhibitor of DNA-binding 2 (ID2), a gene essential for intestinal Peyer’s patches and NALT formation in mice [13] was also upregulated (~7-fold) in the olfactory organ of nasally vaccinated trout compared with controls. CCL19 and ID2 are necessary for the formation and function of NALT in mammals [13] , [14] , [15] . Our findings therefore suggest that CCL19 and ID2 may play a conserved role in the formation and function of NALT in vertebrates. Together, these results may indicate an evolutionary conservation of key NALT-specific molecules from fish to mammals. Histological examination supported the microarray results ( Fig. 5h–k ). At 4 days post immunization (d.p.i.) the olfactory organ of IN vaccinated trout showed a significant enlargement of the LP, increased vascularization and infiltration of neutrophils, macrophages and lymphocytes compared with control or specimens vaccinated by intramuscular (i.m.) injection (the standard delivery mode of IHNV vaccines). By day 14, the tissue reaction was smaller, the LP showed some enlargement and abundant lymphocytes were still present both intraepithelially and in the LP. By day 28, the LP was moderately enlarged but neither myeloid nor lymphoid cells were apparent ( Fig. 5h–k ). The olfactory organs of i.m. injection-vaccinated fish were histologically similar to those of the control group at all time points ( Supplementary Fig. 3 ). Nasal vaccination elicits high protection against aquatic viral diseases The presence of innate and adaptive immune responses in the olfactory organ of rainbow trout following nasal delivery of a viral vaccine led us to test whether nasal vaccination induces protection against pathogen challenge. To the best of our knowledge, nasal vaccines have never been used in aquaculture meaning that this method represents a novel delivery method for the control of aquatic infectious diseases of fish (illustrated in Supplementary Fig. 4a–d ). Because injection vaccination is known to be the most effective vaccination route in fish [16] , and in order to evaluate the efficacy of nasal vaccination, we compared our novel nasal vaccine method (IN) with the well-established i.m. injection delivery (see Supplementary Materials and Methods for details). Our experiments show that nasal vaccination is as effective as the injected vaccine both at early (7 d.p.i.) and late (28 d.p.i.) challenge time points with live virulent IHNV ( Fig. 6 ). These time points reflect the kinetics of innate (7 d.p.i.) and adaptive (28 d.p.i.) immune response of an ectothermic vertebrate such as the rainbow trout. As temperature is such an important factor in the development of adaptive immunity, these challenge points are best defined in degree days (d.d.= T × t ), where T is the temperature in Celsius and t is the time in days. Thus, challenges were conducted at 100 d.d. and 400 d.d. Nasal vaccination was achieved by delivering a 25-μl drop of the vaccine into the left nare of juvenile rainbow trout using a micropipette. Fish were between 3 and 5 g when they receive the vaccine, a standard vaccination size in the salmonid industry. The volume of vaccine deposited into the nare was small enough so that no solution leaked out of the nostril. Fish tolerated the handling and vaccination approach without any apparent problems. Handling times were similar in both the injection and nasal vaccination protocols. We conducted this experiment two independent times (test 1 and test 2) using two different challenge doses of IHNV. In test 1, approximately 40% of the mock-vaccinated control fish died, whereas in test 2, we recorded mortalities of approximately 70%. Both tests revealed the high efficacy of nasal vaccination in rainbow trout. Specifically, IN vaccination conferred 100% and 92–96% protection at 7 and 28 d.p.i., respectively. I.m. injection, in turn, resulted in 88–94% and 91–94% protection at the same time points. 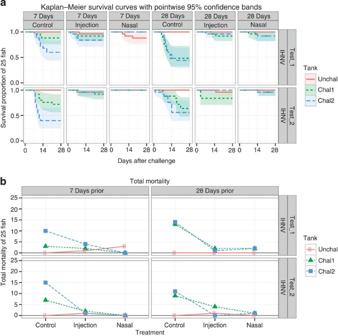Figure 6: Nasal vaccination elicits high levels of protection against infectious haematopoietic virus. Survival curves (a) and total mortality (b) of IHNV intranasal vaccine method (IN) compared with intramuscular (i.m.) injection delivery in two different tests. Trout (N=25 per tank in duplicate tanks) were challenged to virulent IHNV i.p. at 7 and 28 days post vaccination. An exact logistic regression model was used to analyse results as explained in Methods. Chal, challenge; Unchal, unchallenged. Figure 6: Nasal vaccination elicits high levels of protection against infectious haematopoietic virus. Survival curves ( a ) and total mortality ( b ) of IHNV intranasal vaccine method (IN) compared with intramuscular (i.m.) injection delivery in two different tests. Trout ( N =25 per tank in duplicate tanks) were challenged to virulent IHNV i.p. at 7 and 28 days post vaccination. An exact logistic regression model was used to analyse results as explained in Methods. Chal, challenge; Unchal, unchallenged. Full size image Using an exact logistic regression model, we can conclude that there are significant differences between the challenged control group and the two vaccinated challenged groups both in tests 1 and 2. IN vaccination conferred slightly better protection than i.m. injection, although the differences were not statistically significant. Fisher’s exact tests indicate insufficient evidence for differences for nasally vaccinated challenged versus unchallenged ( P -value=1.0); confirming that rainbow trout that received the nasal vaccine had survival rates similar to fish that were not exposed to the virus at all. The complete statistical analysis using the exact regression model and all P -values are shown in Supplementary Table 4 . Nasal vaccination elicits strong protection against aquatic bacterial diseases We next extended the significance of our results by testing a second vaccine, in this case a formalin-killed Yersinia ruckeri bacterin. Owing to the IHNV’s tropism to neural tissues, it may be possible that only live vaccines such as rhabdoviral vaccines are effective when delivered nasally. We chose Y. ruckeri , the causative agent of enteric red mouth disease (ERM), a fatal infectious disease that causes tremendous losses in the aquaculture sector [17] . The ERM vaccine was one of the first vaccines developed for use in aquaculture and is effective by injection and immersion [18] , [19] . We followed a similar approach as in the IHNV model by comparing nasal delivery of ERM to the injection route and measured protection at 7 and 28 d.p.i. following this time a mucosal infection (immersion challenge; Fig. 7 ). Comparing ERM injection to nasal treatments, exact logistic regression shows a treatment-by-challenged interaction with sufficient evidence to conclude that significant differences exist between the challenged control group and all other treatment groups whether challenged or not. At day 7, the survival rate was higher than 92% in both vaccinated groups, whereas the unvaccinated group had a survival rate of 60%. Both vaccine routes conferred 100% protection at day 28. These conclusions are consistent with Fisher’s exact tests of insufficient evidence for differences for the nasally vaccinated and challenged group versus the unchallenged group ( P -value=0.6652), the injection vaccinated and challenged group versus unchallenged group ( P -value=1.0), and the injected vaccinated group versus nasal vaccinated group (both challenged; P -value=0.3687). The complete statistical analysis using the exact regression model and all P -values are shown in Supplementary Table 5 . Altogether, these results indicate that (i) nasal vaccination is also an effective disease control method for use in aquaculture against bacterial diseases; (ii) not only live vaccines but also killed bacterin formulations can be uptaken by the olfactory organ of rainbow trout; (iii) nasal vaccination elicits protection against mucosal infection. 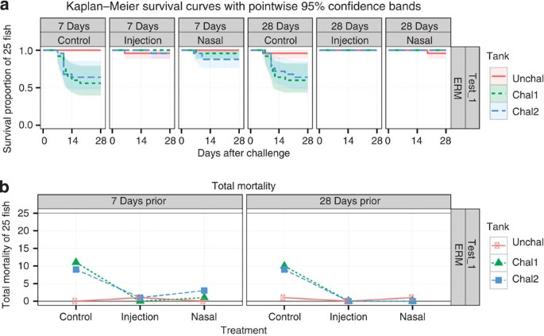Figure 7: Nasal vaccination confers high protection against the bacterial pathogenY. ruckeri. Survival curves (a) and total mortality (b) of ERM intranasal vaccine method (IN) compared with intramuscular (i.m.) injection delivery. Trout (N=25 per tank in duplicate tanks) were challenge (Chal) to virulentY. ruckeriby immersion at 7 and 28 days post vaccination. An exact logistic regression model was used to analyse results as explained in Methods. Unchal, unchallenged. Figure 7: Nasal vaccination confers high protection against the bacterial pathogen Y. ruckeri . Survival curves ( a ) and total mortality ( b ) of ERM intranasal vaccine method (IN) compared with intramuscular (i.m.) injection delivery. Trout ( N =25 per tank in duplicate tanks) were challenge (Chal) to virulent Y. ruckeri by immersion at 7 and 28 days post vaccination. An exact logistic regression model was used to analyse results as explained in Methods. Unchal, unchallenged. Full size image The olfactory system of vertebrates is an ancient sensory system anatomically conserved across species. The present work demonstrates that the vertebrate olfactory system acts far beyond its well-known role as a sensory organ carrying universally conserved defence roles not only in terrestrial but also in aquatic animals. Our findings reveal that early bony vertebrates such as rainbow trout had already developed olfactory organs with defence functions that serve as a primary mucosal immune barrier against pathogens before emergence of terrestrial vertebrates. Here we have shown that teleost NALT follows many of the hallmarks of other teleost MALT. The olfactory epithelium of rainbow trout overall harbours greater numbers of B cells than that of gut and skin but conserves the predominant presence of IgT B cells as well as greater IgT/IgM ratios than in the serum. Our results also underscore the conservation of features between mammalian NALT and teleost NALT despite the absence of organized lymphoid structures (adenoids and tonsils) in teleosts. IgT is the functional equivalent of mammalian IgA [5] . Mammalian secretory IgA (sIgA) plays a crucial role in local defence against bacterial and viral pathogens in the nasal mucosa [20] , [21] and the pIgR is necessary for the presence of sIgA in nasal secretions of mammals [20] , [21] . Similarly, our results suggest a preponderant role of IgT and pIgR in nasal immunity in rainbow trout at the steady state. However, upon nasal vaccination, IgM expression increased to a greater level than IgT in the olfactory organ. At this point, it is unknown whether the same is true at the protein level and whether these Igs are antigen specific. The olfactory systems of vertebrates are characterized by being highly vascularized and therefore present a greater anatomical connection to systemic circulation than other mucosal surfaces. This may result in a very fast recruitment of systemic B cells (dominated by IgM B cells) to the olfactory organ in response to immunization, explaining our results. In addition, cellular immunity such as cytotoxic T-cell responses may be responsible for the protection levels observed, as it is the case in mammals [2] , [22] . Future studies are needed to further ascertain the role of nasal sIg and pIgR as well as cellular immunity in the specific nasal immune responses of teleost fish against pathogens. Another conserved feature between mammalian NALT and teleost NALT is the presence of a symbiotic bacterial community. Here we show for the first time the presence of commensal bacteria in association with the olfactory epithelium of teleosts. Moreover, nasal microbiota appears regulated by trout sIgs as evidenced by the high levels of Ig coating, whereas coating by sIgs has been shown in a number of vertebrate mucosal surfaces. This is the first report that shows that the nasal commensal bacterial community of vertebrates is also controlled by sIgs. In the case of trout nasal bacteria, greater proportions of double-coated and IgM-coated bacteria were found compared with previous gut and skin studies. It is possible that different bacterial communities are present in the olfactory organ compared with the gut and skin and that different Ig isotypes may preferentially coat certain bacterial groups. On the other hand, differences may be attributable to the microbiology of the water that the fish are reared in. In our study, oligomicroarray-based expression studies provided a general view of the biological processes that take place in the olfactory organ of rainbow trout as a result of nasal delivery of a viral antigen. Overall, both innate and adaptive immune molecules are responsive to nasal vaccination. Importantly, these studies have identified NALT-related molecules including adhesion molecules, chemokines and transcription factors known to be crucial in the nasal immune system of mammals. Future studies will address the specific contributions of molecules such as CCL19 and ID2 to the nasal immune responses of teleosts. Here we demonstrate striking protection levels conferred by nasal vaccines against viral and bacterial pathogens of fish. Moreover, protection was achieved against systemic and mucosal challenge to live pathogens. Our findings carry clear implications for the development and implementation of new aquaculture vaccines, a vital aspect to the sustainability and safety of the fish farming industry [23] . As the development of effective fish vaccines in the 1970s, vaccination has been an effective strategy for disease control in aquaculture resulting in millions of fish every year to be immunized worldwide. With a few exceptions, vaccination strategies in aquaculture have remained unchanged over the past 15 years. To date, the most effective route of vaccination used in aquaculture is injection [16] . In addition, mucosal delivery via immersion or oral exposure are used, albeit with generally weaker protective effects [16] . Injection vaccination has some adverse effects to the fish such as granuloma formation, needle use (not amenable to small fingerlings) and requires trained personnel [24] . The immune capabilities present in the teleost olfactory epithelium open up new opportunities for mucosal vaccination of farmed fish via the nares. Based on our studies, control of infectious aquatic diseases, both viral and bacterial, can be effectively achieved by nasal vaccine delivery. We show that nasal vaccination of rainbow trout resulted in systemic protection against IHNV as pathogen challenge consisted of an intraperitoneal (i.p.) injection. Our results are in agreement with numerous mammalian studies where IN vaccination enhances systemic immunity and protects against systemic infection [25] , [26] . On the other hand, in our second vaccine model, ERM, nasal vaccination protected trout from an immersion challenge with Y. ruckeri . Thus, nasal vaccination, similar to in mammals, appears to induce both systemic and mucosal immune responses in teleosts. The exact immune mechanisms by which nasal vaccines confer systemic and mucosal protection in teleosts remain to be investigated. In conclusion, our studies show the widespread and conserved presence of immune functions in association with the olfactory organ of all vertebrates. Thus, it is likely that NALT first appeared as a diffuse lymphoid tissue that protects the olfactory epithelium of aquatic vertebrates against water-carried pathogens and was later adapted towards defence against inhaled antigens. The present work underscores the conserved role of vertebrate olfactory organs in immunity and the emergence of NALT at least 380 million years ago with the appearance of bony fish. Animals Adult specimens (triploid female fish, mean weight=200–300 g) used for flow cytometry, fluorescent microscopy, nasal mucus studies and nasal bacteria isolation were obtained from the Lisboa Springs Hatchery. Goldfish ( C. auratus ) were purchased from a local pet shop, New Zealand groper ( P. oxygeneios ) were obtained from the National Institute of Water and Atmospheric Research and Australian eel ( A. australis ) samples were kindly provided by Dr Mark Lokman (University of Otago, New Zealand). At least three individuals from each species were examined. All rainbow trout used in vaccination trials and microarray studies were obtained from Clear Springs Foods Inc. Vaccination Vaccination experiments were conducted using two different vaccine models: an IHNV live attenuated viral vaccine [27] and an ERM bacterin [28] . Vaccination trials and challenge to live pathogens are described in Supplementary Materials and Methods. All animal procedures were approved by the University of New Mexico IACUC. Collection of serum, olfactory tissue, nasal mucus and nasal bacteria Adult rainbow trout were anesthetized with MS-222, and serum was collected by centrifugation for 15 min at 4 °C, 10,000 g . Trout nasal mucus was gently scraped from the olfactory rosette surface, transferred into an Eppendorf tube, vigorously vortexed and centrifuged at 400 g for 10 min at 4 °C to remove any trout cells present. To separate the nasal-associated bacteria from the mucus, the cell-free supernatant was thereafter centrifuged at 10,000 g for 10 min. The resulting supernatant (nasal mucus free of bacteria) was harvested, filtered with a 0.45-μm syringe filter (Millipore) and stored at −80 °C, whereas the pellet (containing nasal-associated bacteria) was washed three times with PBS (pH 7.2) and resuspended for further analysis. As positive controls, gut- and skin-associated bacteria and mucus were also collected as explained elsewhere [5] , [6] . In addition, blocks of olfactory tissue (both rosettes) were collected and cryoblocks were made using Optimal Cutting Temperature medium (Tissue-Tek). Histology, light microscopy and immunofluorescence microscopy studies The olfactory organs of rainbow trout, goldfish, New Zealand groper and Australian eel were dissected and processed for routine histology. The olfactory organs of control, IHNV vaccinated (IN) and IHNV vaccinated (i.m.) rainbow trout ( N =5–6) were also dissected. All tissue samples were fixed in neutral buffered formalin, paraffin embedded, sectioned and stained with haematoxylin/eosin. Samples were collected at days 4, 14 and 28 post vaccination. Images were acquired in a Zeiss Axioscope microscope using the Axiovision software. Immunofluorescence staining was performed on cryosections obtained from the olfactory organ of adult trout (300 g mean weight). Cryosections were fixed for 3 min in 10% (vol/vol) neutral buffered formalin. Background autofluorescence was eliminated by treatment of cryosections for 10 min with 0.1 M glycine, pH 2.3. For detection of IgT + and IgM + cells, cryosections were incubated overnight at 4 °C with rabbit anti-trout IgT (0.2 μg ml −1 ), mouse anti-trout IgM (IgG1 isotype; 1 μg ml −1 ) or their isotype controls. For the detection of pIgR, cryosections were incubated with rabbit anti-trout pIgR (1 μg ml −1 ). After being washed three times with PBT (PBS containing 0.2% (vol/vol) Triton X-100 and 0.5% (wt/vol) BSA, pH 7.2), samples were incubated for 2 h at 20 °C with indocarbocyanine-conjugated donkey anti-rabbit IgG (711-165-152), indodicarbocyanine-conjugated goat anti-mouse IgG1 (115-175-205; 2.5 μg ml −1 each; all from Jackson Scientific). Nasal-associated bacteria were stained with anti-trout IgM or anti-trout IgT (1 μg ml −1 each), or their respective isotype controls (Biolegend; 2.5 μg ml −1 each), at 4 °C for 1 h with continuous agitation. Skin and gut bacteria were used as positive controls for the experiment. After washing three times, secondary antibodies were added and incubated for 45 min at 4 °C. Before mounting, all samples were stained with DAPI (4,'6-diamidino-2-phenylindole; 1 μg ml −1 ; Invitrogen) for the cryosections or DAPI and Hoechst 33342 dye (5 μg ml −1 each, Molecular Probes) for the bacterial samples. Bacterial samples were cytospun on glass slides and mounted with fluorescent microscopy mounting solution. Images were acquired and analysed with a Nikon Ti fluorescence microscope and the Elements Advanced Research Software (version 4.0). Quantification was performed by two different researchers by counting coating levels in 13 different fields at × 60. Isolation of trout NALT and HK leukocytes For flow cytometry studies, NALT leukocytes (5 × 10 5 ) were isolated by adapting a trout GALT leukocyte isolation method as explained by Zhang [5] . Briefly, leukocytes from trout olfactory organ were obtained by means of mechanical agitation of both olfactory rosettes in DMEM medium (supplemented with 5% FBS, 100 U ml −1 penicillin and 100 μg ml −1 streptomycin) at 4 °C for 30 min. Leukocytes were collected, and the aforementioned procedure was repeated four times. Thereafter, the olfactory organ pieces were treated with PBS (containing 0.37 mg ml −1 EDTA and 0.14 mg ml −1 dithiothreitol) for 30 min followed by enzymatic digestion with collagenase (Invitrogen, 0.15 mg ml −1 ) for 2 h at 20 °C. HK leukocytes were isolated as explained elsewhere [29] and used as a positive control for flow cytometry staining. All cell fractions obtained the olfactory organ following the mechanical and enzymatic treatments were pooled, washed with modified DMEM and layered over 51/34% discontinuous Percoll density gradients. After 30 min of centrifugation at 400 g , cells lying at the interface of the gradient were collected and washed with modified DMEM. Cell suspensions were counted in a haemacytometer. SDS–PAGE, western blot and flow cytometry Nasal mucus and serum samples were resolved on 4–15% SDS–PAGE Ready Gel (Bio-Rad) and analysed by western blot as described previously [5] . Immunoblots were scanned using a ChemiDoc XRS+ System (Bio-Rad) and band densitometry was analysed with Image Lab Software (Bio-Rad). Leukocyte suspensions were double-stained with monoclonal mouse anti-trout IgM an anti-trout IgT (1 μg ml −1 each) on ice for 40 min. APC-rat anti-mouse IgG1 (eBioscience) and PE-goat anti-mouse IgG2b (Santa Cruz Biotechnology) were used as secondary antibodies to detect IgM + and IgT + B cells, respectively. After washing three times, secondary antibodies PE-goat anti-mouse IgG1 or APC-goat anti-rabbit IgG were added and incubated for 45 min at 4 °C. Analysis of leukocytes was performed with an Attune Flow Cytometer (Life Technologies) and Attune software. Fluorescent in situ hybridization Olfactory organ cryosections from adult control rainbow trout were stained with 5′-end-labelled indodicarbocyanine-labelled EUB338 and indodicarbocyanine-labelled NONEUB (control probe complementary to EUB338) oligonucleotide probes (Eurofins MWG Operon). EUB targets the 16S rRNA of ~90% of all eubacteria. Details on oligonucleotide probes are available at probeBase [30] . Hybridizations were performed at 37 °C for 14 h with hybridization buffer (2 × SSC/50% formamide) containing 1 μg ml −1 of the labelled probe. Slides were then washed with hybridization buffer without probes followed by two more washes in washing buffer (2 × SSC) and two washes in PBS at 37 °C. Nuclei were stained with DAPI (5 ng ml −1 ) solution for 25 min at 37 °C. Slides were mounted with fluorescent mounting media and images were acquired and analysed with a Nikon Ti fluorescence microscope and the Elements Advanced Research Software (version 4.0). RNA isolation and quantitative real-time PCR (qPCR) analysis RNA was extracted by homogenization in 1 ml TRIZol (Invitrogen) using tungsten carbide beads (3 mm, Qiagen) and shaking (300 times per min) following the manufacturer’s instructions. The RNA pellet was washed in 500 μl 80% ethanol, air dried and resuspended in RNase-free H 2 O. The concentration was determined by spectrophotometry (Nanodrop ND1000, LabTech) and the integrity of the RNA was determined by electrophoresis (Agilent Bioanalyser, 2100). The RNA was then stored at −80° until required. cDNA was synthesized as previously described [31] . The qPCRs were performed in triplicate and each contained 3 μl of a diluted cDNA template (4 ng of total RNA equivalents), 12.5 μl of Power SYBR Green PCR master mix (2 × ; Applied Biosystems) and 150 nM forward and reverse primers in a 25-μl reaction volume. The amplification profile consisted of an initial denaturation step at 95 °C for 10 min, and then 30 cycles of 95 °C for 15 s and 60 °C for 1 min followed by melting (dissociation stage) from 72 to 95 °C in an ABI Prism 7000 (Applied Biosystems) sequence detection system. A negative control (no template) reaction was also performed for each primer pair. A sample from the serial dilution was run on a 2% agarose gel and stained with Red Gel Stain and viewed under ultraviolet light to confirm a band of the correct size was amplified. A melting curve for each PCR was determined by reading fluorescence at every degree between 72 and 95 °C to ensure only a single product had been amplified. Trout elongation factor EF-1α was used as control gene for normalization of expression. The relative expression level of the genes was determined using the Pfaffl method [32] . Efficiency of the amplification was determined for each primer pair using serial tenfold dilutions of pooled cDNA, performed on the same plate as the experimental samples. The efficiency was calculated as E =10 (−1/s) , where s is the slope generated from the serial dilutions, when Log dilution is plotted against ΔCT (threshold cycle number). Primers were designed to have a Tm of 55 °C, and where possible, to cross an exon–exon junction to avoid amplification of genomic DNA. Exon–intron junction sites were determined by comparing cDNA of genes with genomic sequence for orthologous genes from other vertebrates obtained from Ensembl ( http://ensembl.org/ ). Microarray analysis Nasal delivery of the live attenuated vaccine or PBS into the olfactory cup was performed as described in the Vaccination trial section. Mean weight of trout for these studies was ~5 g. Microarray experiments were performed using a custom-designed, Agilent-based microarray platform with 4 × 44 K probes per slide. The oligos were derived from rainbow trout EST tentative contigs from Rainbow Trout Gene Index Release 7.0 (July 2008); these oligo that were designed by the Dana-Farber Cancer Institute (DFCI) were 70 bases in length, to allow them to be used for Agilent 60 mer platform, the first and last 5 bases of each oligo were removed leaving the ‘mid 60’ nucleotides. 40,125 oligos were from this source. These oligos were supplemented with other immune-related transcripts from more recent releases to National Center for Biotechnology Information and were designed by using the Agilent e array oligo design software (1,287 oligos). These were printed multiple times to fill up the microarray. A further 1,417 Agilent in house control features were included. The array was printed as a randomized design on 4 × 44 K Agilent platform (full details for array platform are available from EBI array express ( http://www.ebi.ac.uk/arrayexpress/ : ‘Trout_imm_v1’_(Agilent array design 028918)) with platform accession A-MEXP-2315. For microarray analysis, four pools of RNA (three fish were pooled due to the small size of the samples) were produced for each time point (4 and 14 days post immunization) from fish that had received a drop of PBS or a drop live attenuated IHNV vaccine into their left nare. Each RNA pool was an equimolar RNA mix from two different fish chosen randomly from each group. The microarray hybridization was performed using a reference RNA sample as previously described [33] . After these relatively stringent procedures, 39,095 of the original 43,730 array features were maintained for subsequent analyses. The experimental hybridizations are at European Bioinformatics Institute archived under accession number E-MEXP: E-MTAB-1812. GO analysis Enrichment for GO biological processes was performed on all cDNA features that had GO identifiers associated using the GOEAST programme [34] . Fisher’s exact test was performed within the GOEAST programme to determine whether GO identifiers occurred more often in a group than would appear by chance. For GO analysis, only biological process GO identifiers were considered that occurred more than three times. For microarray analysis, fold change differences between control and IHNV-injected samples were calculated using cutoff of twofold. Significant differential expression at each time point (4 and 14 d.p.i.) was established by two sample (unpaired) t -test ( P <0.05) with unequal variance. The Benjamini–Hochberg false discovery rate correction within Genespring software was applied. The qPCR measurements were analysed by the unpaired t -test, with P -values <0.05 considered significant. All the expression data are presented as mean±s.e. Vaccination trials Two separate vaccine trials (IHNV test 1 and IHNV test 2) were conducted with an attenuated vaccine made against IHNV. The virus was originally isolated in cell culture from a clinically diseased rainbow trout obtained from a private fish farm located in the Hagerman Valley, Idaho, using standard methods. This IHNV isolate was attenuated by serially passing it over 100 × in a Chinook salmon embryo-214 cell line. In both vaccine trials, 150 fish groups of specific pathogen-free rainbow trout (mean weight, 4 g for the first trial and 6 g for the second trial) were immunized by pipetting 25 μl into the right nare (IN) or by injecting 25 μl i.m. into the dorsal musculature just anterior to the dorsal fin of attenuated IHNV suspension that contained 1 × 10 6 plaque-forming units (PFU) ml −1 . A mock immunized group received 25 μl of cell culture media (MEM-2) both IN and i.m. without the attenuated virus. Duplicate 25-fish groups from each treatment were challenged with IHNV at 7 (100 d.d.) and 28 (400 d.d.) d.p.i. Briefly, fish were anaesthetized in MS-222 and injected with IHNV isolate 220-90 (ref. 35 ). In the first test, fish were injected i.p. with 5 and 100 PFU at 7 and 28 d.p.i. at mean fish weights of 5 and 11 g , respectively. In the test 2, fish were injected with 5,000 and 10,000 PFU at 7 and 28 d.p.i. at mean fish weights of 7 and 13 g, respectively. An additional 25-fish group from each treatment was mock challenged by injecting cell culture media without virus at each challenge interval. After viral challenge, each 25-fish group was held in separate 19 l aquaria that received flow through 15 °C ultraviolet light-treated spring water and monitored for mortalities for 21 days. A minimum of 20% of the fish that died on any given day were tested for IHNV by plaque assay. Relative percent survival was calculated using the following formula: (1–% mortality of vaccinated fish/% mortality of control fish) × 100. At 7–8 weeks post immunization, fish from each group were euthanized with a lethal dose of MS-222, and bled to test for IHNV neutralizing antibody titres. A vaccine trial was conducted with a formalin killed Y. ruckeri ERM bacterin. The ERM test compared i.p injection with nasal delivery. Groups of 140 specific pathogen-free rainbow trout (mean weight, 7 g) were immunized by pipetting 25 μl IN of a 1:10 dilution of the stock vaccine (2 × 10 9 CFU ml −1 ) or by injecting i.p. 25 μl of the same vaccine. A mock-immunized group received 25 μl of saline (0.85%) both IN and i.p. Y. ruckeri bacteria used for the challenge were grown on tryptic soy agar (TSA) for 48 h at 15 °C. The bacteria were harvested by adding 5 ml of saline to the TSA plates. The concentration of the bacteria was calculated by measuring absorbance at 640 nm, which corresponded to a bacterial suspension of 5 × 10 8 CFU ml −1 . Fish from each treatment group were challenged by immersion in a total volume that was 10 × the total weight of the fish in grams with 100 and 200 ml of the 50% bacterial suspension at 7 and 28 d.p.i. Mean fish weights at these times were 9 and 17 g, respectively. Challenges were conducted statically for 1 h with air added to the tank. Fish were placed in 19 l flow through aquaria after the challenge period. An additional 25-fish group from each treatment was mocked challenged by exposing the fish to water only. A minimum of 20% of the fish that died on any given day were tested for Y. ruckeri by culturing kidney tissue on TSA. Relative percent survival was calculated and comparisons between treatments made. Statistical analysis of vaccination trials: exact logistic and Fisher’s tests Exact logistic regression [36] using SAS [37] models the log odds of the binary outcome of mortality of each of 25 fish within 28 days of either an IHNV or an ERM pathogen challenge as a linear combination of main-effects and interactions of the predictor variables: number of days from vaccination to pathogen challenge (7, 28), which treatment (control, injection, nasal), whether pathogen challenged (challenged, unchallenged), tank number (for replicated challenge treatments) and test number (when entire test was pseudo-replicated). Regular logistic regression using the standard maximum-likelihood-based estimator is unreliable for analysing small, skewed or sparse data sets, such as when some responses for combinations of categorical predictor variables have no observations. The estimates given by exact logistic regression do not depend on asymptotic results. A final model for the mortality dependence pattern observed for each experiment was chosen using backward selection starting with a full first-order model up to three-way interactions. Fisher’s exact test of conditional independence for a two-dimensional contingency table is used to test specific a priori contrasts between treatment and challenge groups [38] , [39] . IHNV tests 1 and 2: injection versus nasal Although survival characteristics differed for IHNV between the two tests and two replicate tanks, the same general pattern is supported. Treating the reference group as the 28 days challenged injected vaccinated group, the final model includes an interaction for treatment and challenge, as shown is Fig. 5 . With our choice of reference group, the parameter estimate table indicates sufficient evidence to conclude differences between the challenge control group from the other challenged treatment groups, that is, there is insufficient evidence to conclude differences between injection and nasal treatment challenged groups ( Supplementary Table 4 ). Furthermore, Fisher’s exact tests indicate insufficient evidence for differences for nasal: challenged versus unchallenged ( P -value=1.0) and marginal evidence for differences for challenged: injection versus nasal ( P -value=0.04615) with nasal having slightly less mortality. ERM test: injection versus nasal Treating the reference group as the 28 days challenged injection vaccinated group, the final model includes an interaction for treatment and challenge. With our choice of reference group, the parameter estimate table indicates sufficient evidence to conclude differences between the challenged control group from all other groups, that is, there is insufficient evidence to conclude differences between injection and nasal vaccine treatment groups whether challenged or not and the unchallenged control group ( Supplementary Table 5 ). Other statistical analyses Data were analysed in Prism version 5.0; GraphPad. Data are expressed as mean± s.e. Unpaired t -tests were used for analysis of differences between groups. P values less than 0.05 were considered statistically significant. How to cite this article: Tacchi, L. et al. Nasal immunity is an ancient arm of the mucosal immune system of vertebrates. Nat. Commun. 5:5205 doi: 10.1038/ncomms6205 (2014).